Density functional theory calculations of continuum lowering in strongly coupled plasmas An accurate description of the ionization potential depression of ions in plasmas due to their interaction with the environment is a fundamental problem in plasma physics, playing a key role in determining the ionization balance, charge state distribution, opacity and plasma equation of state. Here we present a method to study the structure and position of the continuum of highly ionized dense plasmas using finite-temperature density functional theory in combination with excited-state projector augmented-wave potentials. The method is applied to aluminium plasmas created by intense X-ray irradiation, and shows excellent agreement with recently obtained experimental results. We find that the continuum lowering for ions in dense plasmas at intermediate temperatures is larger than predicted by standard plasma models and explain this effect through the electronic structure of the valence states in these strong-coupling conditions. The recent development of free-electron lasers (FELs) operating in the X-ray regime, such as the Linac Coherent Light Source (LCLS) in the USA [1] and SACLA in Japan [2] , is providing new ways to study highly ionized and dense plasmas with unprecedented accuracy and control. The intense, femtosecond-duration pulses that can be generated at X-ray wavelengths at such facilities are of interest since thin foils can be driven to highly excited, high-temperature conditions isochorically on inertially confined timescales, opening the way for the study of warm- and hot-dense plasmas in well-defined conditions of density and temperature. A recent experiment reported heating Al plasmas to temperatures between 100 and 200 eV in <80 fs, that is, on timescales so short that no significant ion motion could take place, removing any relevant experimental uncertainty on the ion density of the plasma studied [3] . Given that the predominant FEL–matter interaction channel was K-shell photoabsorption, the tracking of ionization, electron density and energy deposition could be performed in a relatively straightforward way via an atomic-kinetic calculation, providing a reliable handle on electron density and, to a slightly lesser degree temperature, all as a function of time. These well-defined plasmas were studied using K α emission spectroscopy, and provided an experimental determination of the K-edge positions for a range of ionic charge states in a dense, strongly coupled plasma for the first time [4] . Since the electron temperatures and densities were known to a good precision, the plasma ionization potential depression (IPD) could be extracted from the measurements by comparing with known atomic edges, as a function of the ionic charge state. Importantly, since the experiment does not rely on recombination from the continuum, these results are not limited by the well-known problem of line broadening as the spectroscopic series merges into the continuum. The importance of such experiments lies in their ability to provide accurate and unique experimental data that can be used to benchmark assumptions, models and codes commonly used within the plasma physics community, yet which have never been rigorously tested in many of the conditions in which they are often employed. In particular, the influence of the surrounding plasma on an embedded ion—which leads to a depression in its ionization potential—is essential to determine plasma properties such as the energy balance, charge state distribution (CSD), equation of state and opacity, yet is notoriously difficult to measure accurately. Accounting for the change in ionization potentials in ions due to plasma effects is important in all but the hottest dilute plasmas. Analytical models are popular as they provide a conceptually simple physical basis for the lowering of the ionization energy, are relatively straightforward to implement in codes and are computationally efficient. The simplest such approach is the ion sphere (IS) model, assuming a constant free-electron density within a Wigner–Seitz IS [5] , [6] . This model is based on condensed matter theory and is generally considered valid only at low temperatures and high densities. At the opposite extreme, at high temperatures and low densities, the Debye–Hückel theory is applicable and the IPD can be evaluated in terms of the Debye screening length [7] . One of the most popular analytical models for the IPD is that due to Stewart and Pyatt (SP), which bridges between the IS and Debye–Hückel results, and is therefore used over an extended range of plasma conditions [8] . Another model that is thought to be applicable over an extended range of temperatures and densities, albeit with different expressions, is that due to Ecker and Kröll (EK) [9] . This model has gained some popularity of late [10] , [11] , as a modified version of this IPD (but using the same screening length) has been shown to agree well with experimental measurements in dense plasma conditions on LCLS [4] . Further information on these analytical models, and on their applicability to the study of dense plasmas, can be found in ref. 12 . Models accounting for the IPD in a plasma need not be analytical. The ionization potentials can be calculated by treating the effect of the surrounding plasma on the ions directly, so that an external model for the IPD is not required, such as in the average-atom approach of Crowley [13] . First-principle calculations based on density functional theory (DFT) also account for IPD-type effects in a self-consistent way and do not necessitate external IPD corrections [14] . The success of various models must be gauged by comparing them with experimental observations. The recently reported experimental determination of the IPD in dense Al plasmas via K-edge measurements on LCLS [4] cites a large discrepancy between the experimental result and the predictions based on the SP or IS models. In contrast, a modified model based on EK was found to agree very well with the experimental data, unfortunately however, without providing any particular physical insight into why this might be so. More recently, Hoarty et al. [15] have constrained the possible values of the IPD in Al plasmas heated to temperatures in excess of 500 eV, and over a range of ion densities, using very thin Al foils embedded in plastic or diamond, compressed and heated by the Orion laser at AWE. Their results agree qualitatively with the predictions of SP, and are inconsistent with the EK model for the temperatures and densities they quote to have reached. Bearing in mind that although the LCLS and AWE experiments were conducted in moderately different plasma coupling conditions, the two models still remain mutually incompatible [12] , [15] , and the large continuum lowering observed in the LCLS experiments has proven challenging to explain with existing models. In this paper we present electronic structure calculations for an Al ion of given charge state Z immersed in a dense plasma at finite temperatures using ab initio DFT. We calculate the K-edge energies for these ions over a range of temperature, electron density and CSD conditions within a truly multi-centred model, going beyond the average-atom approach, and compare our results with recent experimental data from LCLS [4] . Set-up of the calculation We have employed the finite-temperature plane-wave DFT code ABINIT [16] , [17] , [18] to calculate electron states and energies within a plasma, in combination with the projector augmented-wave (PAW) potential formalism [19] , [20] , [21] used to model a range of different Al ions. The highly charged ions needed for plasma charge state calculations are constructed by creating excited-electron configurations in inner atomic shells and freezing them in the core of the potential. The use of excited potentials in DFT calculations to study the electronic structure, often investigated experimentally by photoemission spectroscopy, is an established technique [22] , [23] , [24] , [25] , and has been recently adapted to the frozen-core PAW formalism to study the properties of dense plasmas [26] . This technique has since been successfully applied to interpret XANES measurements on dense Al plasmas with a 1 s core hole [27] , and to the study of X-ray emission spectroscopy and electronic structure of L-shell-excited Al on the VUV FEL FLASH [28] . Our calculation proceeds as follows. We start by constructing PAW potentials to be used in the DFT calculation with the K and L-shell electrons (1 s , 2 s and 2 p states) frozen in the core [29] . These states are frozen in the sense that they cannot be relaxed, depopulated or changed in the subsequent DFT calculation and represent the ion-core, or ion charge state. For aluminium, the lowest meaningful charge state that can be generated in this manner is Z =3, corresponding to placing the atomic 3 s and 3 p electrons in the valence states, which then constitute the metallic bands of Al in the low-temperature solid-state limit. From the plasma physicist’s point of view these electrons lie in the continuum of states. Increasingly higher charge states are subsequently generated by removing electrons from the 2 p , and later 2 s atomic states, and placing them in some higher M-shell orbital. These electrons remain in the system—which is therefore charge neutral by construction—and will end up populating the continuum states in such a way as to minimize the total free energy. We note that imposing charge neutrality here is a choice rather than a limit, and one could equally well create truly ionized configurations for which the system would be globally charged. Given that we are ultimately guided by the experimental results, charged systems will not be considered in what follows. Once generated, the PAW potentials are used in a plane-wave DFT calculation for an extended system modelled via a cubic supercell with periodic boundary conditions. The structure of all the electrons not frozen in the core via the PAW potential is obtained by solving the finite-temperature Mermin–Kohn–Sham effective Schrödinger equation, yielding the self-consistent valence wavefunctions, eigenvalues and occupation factors. These solutions represent the equilibrated effect of the environment on the plasma ions: the DFT calculation finds the finite-temperature ground-state solution for all the valence electrons subject to the given ionic potentials, which contain the desired configurations of ionized core states. Because of this, the temperature and the ionic charge state are independent quantities in our calculations. Importantly, since the PAW potentials contain all relevant information on the core wavefunctions, the total internal energy of the system—valence, core and interaction—can be computed, as can the valence electron density and the local projected density of states (pDOS) within a sphere centred on a specific atom. Electron density and charge state dependence The calculated continuum DOS is shown in Fig. 1 for a set of ionic configurations, at an electron temperature of 1 eV. The simulation is conducted for a face-centred cubic Al unit cell containing four ions, one of which is ionized seven times (that is, with four core holes in the 2 p state), while the other three ions vary in charge state between 3+ and 11+, representing ions ranging from a completely full to a completely vacant L-shell. The DOS of the full system, as well as the pDOS local to the 7+ ion are shown. The zero-energy level is that of the corresponding isolated ionic potential, from which atomic-like core-bound state energies are measured. As the charge states increase, so does the electron density in the system, starting at 2.4 × 10 23 cm −3 and reaching 6.0 × 10 23 cm −3 for the 11+ configuration. We note a clear systematic change in both the structure and the position of the continuum with density. 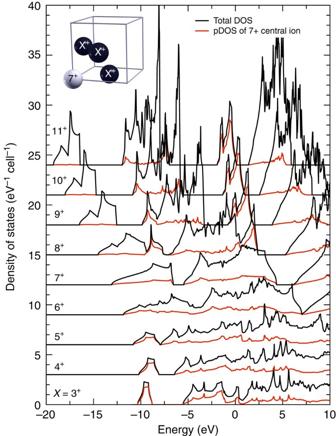Figure 1: Valence DOS for a range of charge state configurations. Total DOS of an Al face-centred cubic (FCC) cell containing a 7+ ion surrounded by different environments at a temperature of 1 eV. The local pDOS of the 7+ ion is shown illustrating the states available to that ion compared with the total system. Initially, the 7+ ion exhibits a broad atomic 3s-like state that is subsumed into the continuum as the total density increases. Figure 1: Valence DOS for a range of charge state configurations. Total DOS of an Al face-centred cubic (FCC) cell containing a 7+ ion surrounded by different environments at a temperature of 1 eV. The local pDOS of the 7+ ion is shown illustrating the states available to that ion compared with the total system. Initially, the 7+ ion exhibits a broad atomic 3 s -like state that is subsumed into the continuum as the total density increases. Full size image The number of atoms that can be treated by this calculation is somewhat limited; here we have used supercells containing up to 32 atoms. For the purpose of this work we deem this number sufficient; however, for a more detailed study of CSD effects or of more exotic structures, larger supercells can and should be used. For the one- and four-atom cells a perfect crystal structure is assumed that considerably simplifies the calculations given the many symmetries that can be exploited in sampling the Brillouin zone. This has been particularly beneficial in the high-electron-temperature calculations for which the necessary number of bands required for a converged calculation becomes quickly prohibitive with an increasing number of electrons. The larger 32-atom cells allow us both to test the convergence due to box size of the smaller calculations, as well as to include some deviation from the ideal crystallographic positions based on the physical temperature of the lattice by using molecular dynamics; if the system under study contains cold ions this effect will be overall small, simply washing out some of the more pronounced features in the DOS. However, if the ions are hot, a crystallographic calculation is no longer representative and large cells with full molecular dynamics are needed. In the following we will be interested in comparing our calculations with the experimental results obtained on LCLS [3] , [4] , where the femtosecond nature of the X-ray pulse guarantees the ions remain relatively cold during the measurement. We have nevertheless estimated the effect of a thermal lattice compared with the ideal crystal by determining the position of the atoms in a 32-atom supercell via a ground-state DFT calculation coupled to molecular dynamics using the Verlet algorithm with a Nose–Hoover thermostat thermalized to temperatures between 300 and 1,000 K. No significant effects on the results presented were observed. Electron temperature dependence To study the effect of temperature on the continuum structure we have chosen a specific charge state configuration in a four-atom supercell—a single ion of charge 7+ surrounded by 6+ ions—which was investigated for a range of temperatures between 1–100 eV. The mean electron density for this configuration is 3.75 × 10 23 cm −3 . Our results, shown in Fig. 2 , illustrate the continuous process of formation of atomic lines from the continuum: these lines are initially broad but become increasingly peaked towards the atomic value as the temperature is increased. At the highest temperatures investigated we have observed the formation of a quasi-atomic 3 s line, as well as the onset of formation of atomic-like 3 p features. This observation of the tendency to form atomic-like states at higher temperatures is encouraging in the context of the observation of bound n =3 states of He-like Al in the AWE Orion experiments, but the clear lack of such bound states in the lower-temperature LCLS data. We note that the EK model, which agrees well with the LCLS data, predicts that the M-shell never rebinds at or above solid density [12] , which places it in stark contrast with the observed experimental results on Orion and with the calculations presented here. 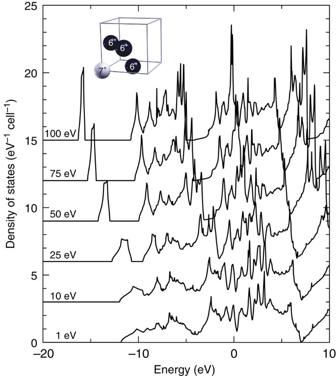Figure 2: Valence DOS for a range of temperatures. Total DOS of an Al FCC cell containing a 7+ ion surrounded by 6+ ions at different temperatures. The line that emerges at the lowest energies at high temperature corresponds to the atomic-like 3sstate on the 7+ ion. Figure 2: Valence DOS for a range of temperatures. Total DOS of an Al FCC cell containing a 7+ ion surrounded by 6+ ions at different temperatures. The line that emerges at the lowest energies at high temperature corresponds to the atomic-like 3 s state on the 7+ ion. Full size image Within the context of determining the charge state of the ion we emphasize that while some states tend to the atomic limit they still retain some level of delocalization at all temperatures investigated and are in any case only weakly populated. For the 7+ ion at 75 eV we find that the population of the 3s -like peak shown in Fig. 2 is <0.18, while at 100 eV it is 0.12 electrons, so that even if considered fully bound, the change in core charge state would be small. Importantly, because our DFT results treat bound, semibound and continuum states in exactly the same manner, even such detailed effects remain fully accounted for in our calculations of the theoretical K-edge and do not impact our comparison with experimental data. Our observation of no significant rebound electron density in the valence states is further consistent with the experimental results from LCLS, which also found no evidence for atomic M-shell states, as well as with the analytical models [4] . We conclude that for the conditions investigated we may describe the ionic charge state by the K- and L-shell populations alone. The shift in the position of the continuum as a function of temperature can again be estimated from these results in much the same way as was done previously for a varying CSD and, consequentially, electron density. We note from Fig. 2 that the energy at which we start to observe continuum states in the DOS changes very little with temperature. Further, although the distinction between continuum states and localized, rebinding states is blurred at finite temperatures (so that a precise definition of what constitutes a bound and what a free state depends somewhat on nomenclature), the uncertainty in energy this might introduce is at most ~5 eV. Given the experimental uncertainty in the determination of the K-edge of ~20 eV (ref. 4 ), we shall neglect such detailed accounting in the present discussion. Although the electron DOS does not vary dramatically with temperature, the population of electronic states will change significantly as the temperature is raised up to 100 eV. To show the temperature effect on the electron density distribution we plot in Fig. 3 the radial electron density surrounding an Al 7+ ion for the same CSD and at the same temperatures shown in Fig. 2 . As can be seen from Fig. 3 , when the system is cold the electron density within half a Bohr radius of the nucleus strongly resembles that of the isolated neutral atom in an excited configuration with seven electrons in the M-shell. As the temperature rises the densities become increasingly more homogeneous and the value of the density outside the immediate ion core slowly tends to the mean density (that is, the value that would be obtained assuming a perfectly homogeneous free-electron gas). Nevertheless, the electron density is seen to remain consistently above this average value at all temperatures investigated. 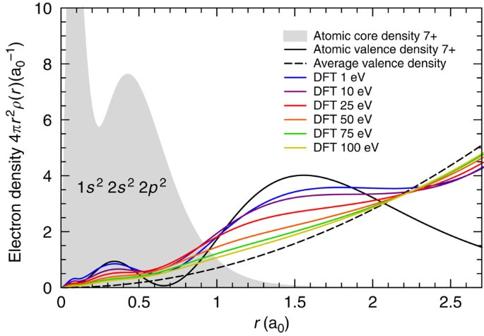Figure 3: Radial electron density of a 7+ ion at different temperatures. Comparison of radial electron densities as a function of temperature within a sphere of radius equal to half the nearest neighbour distance (2.7 Bohr radii) centred on an Al 7+ ion, in an FCC lattice surrounded by 6+ ions. Also shown is the core (K- and L-shell) and the valence (M-shell) electron density for an isolated Al 7 times excited atom, and the electron density assuming a completely homogeneous distribution for all the free electrons within the simulation volume (25 electrons per four-atom unit cell). Figure 3: Radial electron density of a 7+ ion at different temperatures. Comparison of radial electron densities as a function of temperature within a sphere of radius equal to half the nearest neighbour distance (2.7 Bohr radii) centred on an Al 7+ ion, in an FCC lattice surrounded by 6+ ions. Also shown is the core (K- and L-shell) and the valence (M-shell) electron density for an isolated Al 7 times excited atom, and the electron density assuming a completely homogeneous distribution for all the free electrons within the simulation volume (25 electrons per four-atom unit cell). Full size image To compare our results with the measured IPDs from the LCLS experiments, we proceed to extract the theoretical plasma K-edges from the DFT calculations. We do this by calculating the difference in total free energy (for example, see Kraisler et al. [30] ) between a system with and without a single K-shell hole, in the presence of a given number of additional L-shell holes. The electron removed from a K-shell is placed in a valence state and is equilibrated in the DFT calculation, so that overall charge neutrality of the systems is preserved. The calculated energy difference yields the total amount of energy needed to transit between the two configurations at a some given, fixed, temperature. However, since the two DFT calculations that are being compared are individually in thermal equilibrium, the energy difference between the two is not equal to the K-edge alone, which we define for a photoionization process as the energy required to make the transition from the 1 s state to the lowest-energy state in the continuum. This is because clearly some additional energy is required to thermalize the electron excited from the 1 s state with the rest of the electrons in the valence band. It is simple to account for this effect: in the low-temperature limit the additional energy acquired is simply the Fermi energy, while at high temperatures it is given by the mean thermal energy of the valence electrons. For completeness we also note that an accurate determination of the absorption K-edge for a specific atomic configuration requires, in principle, information about the angular momentum properties of the final states, since transitions associated with the absorption of a photon must obey the relevant selection rules. This effect, while tractable within the present treatment, is negligible for the systems discussed here. Our calculated K-edge values are shown in Fig. 4 , compared with the LCLS experimental results on solid-density Al and with the three analytical models mentioned earlier. The agreement between the experimental data and our results is excellent across the entire range of measured charge states. To simplify the comparison, the calculations presented in Fig. 4 are for a CSD containing only a single charge state, and so do not take into account the effect of different charges surrounding the emitting ion. Although not strictly representative of the experiment, a detailed accounting of the local CSD present in the plasma when the K-edge was measured for each ion charge state requires a rather involved treatment of the atomic kinetics—itself IPD-dependent—and is outside the scope of this discussion. This approximation is justified by noting that from the calculations on Al presented in ref. 4 , the mean electron density for all measured ion edges differed by less than one charge state from that of the emitting ion, and that such a small variation in the CSD is seen to have a negligible effect on the position of the K-edge in our calculations (see neighbouring curves in Fig. 1 ). 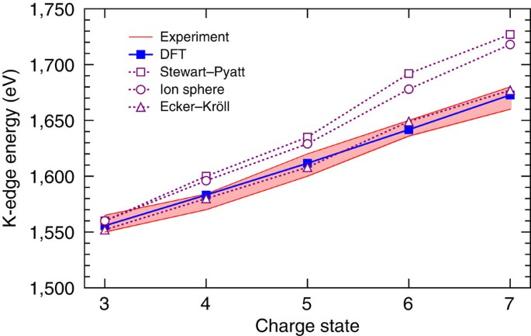Figure 4: Comparison of calculated and experimentally measured K-edge energies in Al. K-edge energies for Al for a range of ion charge states. The band corresponds to the experimentally determined edge positions with errors, as given by ref.4, plotted alongside the SP, EK and IS models. The results from this work are marked DFT. Figure 4: Comparison of calculated and experimentally measured K-edge energies in Al. K-edge energies for Al for a range of ion charge states. The band corresponds to the experimentally determined edge positions with errors, as given by ref. 4 , plotted alongside the SP, EK and IS models. The results from this work are marked DFT. Full size image The DFT K-edge energies shown were calculated for a relatively cool system at 1 eV, but assuming electrons can be excited into the lowest energy state in the continuum, that is, we assume that the temperature distribution of the valence electrons is on the order of the Fermi energy (10–20 eV). As the position of the continuum in the DOS changes very little for all the temperatures considered (see Fig. 2 ) this approach simplifies the calculations considerably without introducing any significant error. We note that a relatively weak temperature dependence of the IPD (at constant electron density) is very important if an IPD model is to be compared with experiment. This is due to the intrinsic difficulties of extracting precise, model-independent temperatures from spectroscopic experimental data. In fact, the authors of ref. 4 provide only an upper limit for these temperatures from their atomic-kinetic calculations, assuming instant thermalization of the valence electrons during the evolution of the FEL-irradiated system and at peak intensity of ~4 eV for charge state Z =3 and 80 eV for charge state Z =7. Importantly, the weak temperature dependence observed is not a particular feature of our calculations: in these conditions the SP model discussed above exhibits a weak dependence, while the IS and EK models have no explicit temperature dependence at all. Of course, both the CSD and the temperature simplifications are ultimately justified by the fact that their combined effect seems to present only a small correction to the position of the continuum, which is in any case smaller than the uncertainties from the experimental measurements. The K-edge may also be extracted from a single DFT calculation by computing the difference between the 1 s binding energy and the energy of the lowest continuum state directly. However, this method is complicated by the well-known problem of obtaining absolute binding energies within the DFT formalism. In fact, the simple isolated atom calculation of ground-state Al yields a 1 s binding energy that is underestimated by ~35 eV, and yields a correspondingly incorrect K α (2 p −1 s transition) energy. To circumvent this issue, the atomic 1 s energies for each charge state can be shifted by the amount required to yield the experimentally known values for the K α energies of that charge state [3] . The required shifts are seen to be between 35–40 eV for all the Al charge states, ranging from 3+ to 11+. These shifted levels may then be compared with the DFT calculated energies of the valence states to yield the theoretical K-edges. In Fig. 5 we show the comparison between the calculated K-edge energies for all charge states in Al that can emit a K α photon using these two methods, again for a system at 1 eV. Excellent agreement is found between the two, to within 0.1–0.2% across the entire charge state range. We have also included, for reference, the K-edge assuming the lowest valence state was available, as used in the comparison with experimental data, which, as mentioned, differs from the above by the Fermi energy. 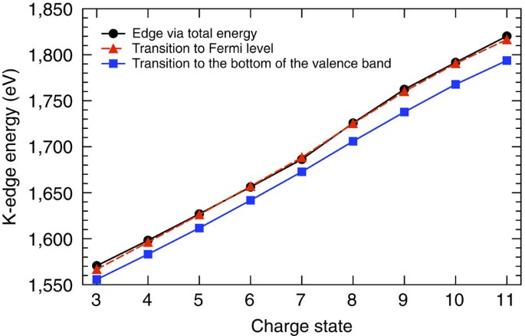Figure 5: Comparison of DFT-determined K-edge energies. The curves for the K-edges correspond to the two different methods described in the text and are calculated for a system at a temperature of 1 eV. Figure 5: Comparison of DFT-determined K-edge energies. The curves for the K-edges correspond to the two different methods described in the text and are calculated for a system at a temperature of 1 eV. Full size image The energy trend of the K-edge positions as a function of charge state, and the weak temperature and average environmental density dependence they exhibit, can be understood in terms of the electronic structure of valence electron states near core-excited ions in strong-coupling conditions. Specifically, we observe that the valence states preserve much of their atomic features, especially at low temperatures, so that the local environment around a given ion is quite different to that suggested by average quantities, as can be seen for electronic densities in Fig. 3 . The implication is that quantum effects such as wave function orthogonality between core and valence electrons should not be neglected in determining electronic states and densities (and hence K-edges), but also that the lowest energy states in the continuum may lie at different energies for neighbouring ions of different charge. This latter point may be observed from Fig. 1 by comparing the onset of the DOS arising from the environmental atoms (denoted by X + and drawn in black) with the DOS local to the 7 + atom (shown in red). Further, we observe that while the electron density does become more homogeneous with temperature, this is predominantly due to the thermal distribution function spreading electrons over an increasingly large number of states rather than due to a strong change in the DOS—the latter, as shown in Fig. 2 , changes very little, leading to a very weak temperature dependence of the K-edge. The importance of accounting for the full quantum mechanical structure of the valence electrons has been recognized in the past and the densities shown in Fig. 3 contain similar features to the valence densities calculated using self-consistent field IS methods [31] . However, our calculation goes beyond such average-atom approaches in that it is a true multi-centred treatment of the plasma environment with no requirement of spherical symmetry, which can compute a fully three-dimensional (3D) electron structure, and from it, the full DOS. While the average electron temperatures and densities are therefore not particularly useful parameters to model our system, atomic state energies in neutral or quasi-neutral atoms are. We find that a relatively good estimate of the K-edge energies in these plasma conditions can be made via simple atomic considerations of inner-shell electron excitation rather than ionization, that is, transition energies of electron excitations between the K and M shells for isolated, excited, yet neutral Al atoms. From this observation it follows that the IPD for a given charge state can be estimated surprisingly well by subtracting the energy of an excited, neutral atom from the corresponding energy required to create an ion with the same K and L shell configuration. This is seen to yield reasonable values for the IPD for all the charge states investigated, as can be quickly verified using available online excitation and ionization codes (for example, see ref. 32 ). Nevertheless, we stress that although this picture may be useful for a quick estimate of the K-edge energies within a few 10’s of eV, an atomic picture for the DOS or electron densities would be incorrect as the valence states are not atomic in nature or localized—except perhaps at the highest temperatures—and a general solution for the position and structure of the continuum still requires a complete DFT calculation. Details of the calculations The DFT calculations presented in this work were conducted using 1-, 4- and 32-atom cells in an face-centred cubic lattice, with a Monkhorst–Pack grid sampling [33] for the k -points ranging between 40 × 40 × 40 (for the results shown in Fig. 1 ), and 12 × 12 × 12 (for the results shown in Fig. 2 ), corresponding to 1,771 and 84 points in the irreducible Brillouin zone, respectively. The DOS calculations presented were all computed using the tetrahedron method. The plane-wave energy cutoff used in the calculations was of up to 1,100 eV, while for the PAW grid a much higher cutoff of 2,700 eV was used to ensure an accurate mapping of the valence electron density close to the atomic cores. The grid resolution allows for a PAW compensation charge convergence of better than 10 −6 . For all calculations the zero-temperature exchange and correlation potentials in the PBE form of the generalized gradient approximation were used [34] . We note that this will introduce a small but systematic error in all our finite-temperature results. Reaching the same energy convergence at finite temperatures well above the Fermi temperature as can be achieved at zero temperature is very challenging, owing to the finite population of high-energy states. This requires a large number of states, or bands, to be considered in the DFT calculation. For our finite-temperature calculations we have ensured we sample electron energies up to at least 10 times the temperature, so that the error on the total energy due to the band-number cutoff does not exceed 0.1%. This corresponds to ~160 bands at 10 eV, 600 at 25 eV, 1,700 at 50 eV, 3,100 at 75 eV and 5,000 bands at 100 eV. These latter calculations can be quite cumbersome; the computational expense of a calculation with 5,000 bands was seen to have been in excess of 4,500 cpu-hours (~190 cpu-days) for a four-atom supercell containing 25 electrons. How to cite this article: Vinko, S. M. et al. Density functional theory calculations of continuum lowering in strongly coupled plasmas. Nat. Commun. 5:3533 doi: 10.1038/ncomms4533 (2014).